Universal epitaxy of non-centrosymmetric two-dimensional single-crystal metal dichalcogenides The great challenge for the growth of non-centrosymmetric 2D single crystals is to break the equivalence of antiparallel grains. Even though this pursuit has been partially achieved in boron nitride and transition metal dichalcogenides (TMDs) growth, the key factors that determine the epitaxy of non-centrosymmetric 2D single crystals are still unclear. Here we report a universal methodology for the epitaxy of non-centrosymmetric 2D metal dichalcogenides enabled by accurate time sequence control of the simultaneous formation of grain nuclei and substrate steps. With this methodology, we have demonstrated the epitaxy of unidirectionally aligned MoS 2 grains on a, c, m, n, r and v plane Al 2 O 3 as well as MgO and TiO 2 substrates. This approach is also applicable to many TMDs, such as WS 2 , NbS 2 , MoSe 2 , WSe 2 and NbSe 2 . This study reveals a robust mechanism for the growth of various 2D single crystals and thus paves the way for their potential applications. The direct synthesis of two-dimensional (2D) single crystals on desired substrates is essential for high-end applications, such as integrated electronic and optoelectronic devices. Among the ~1800 2D materials predicted by high-throughput computation, more than 99.5% have a non-centrosymmetric crystalline structure. During the growth of non-centrosymmetric 2D materials, antiparallel grains are frequently observed because of their energetic equivalency on most substrates [1] , [2] , [3] , [4] , [5] , [6] , [7] , [8] , [9] , [10] , [11] , [12] , [13] , [14] . To break this equivalence, atomic steps on the surface were introduced and proved effective for the epitaxial growth of single-crystal hexagonal boron nitride (h-BN) and transition metal dichalcogenides (TMDs) on a few specially-designed substrates, such as vicinal Cu(110) and a- or c-plane sapphire. Until now, these successes were attributed to two different mechanisms, (i) step-edge-guided epitaxy, namely the edge-docking mechanism, and (ii) epitaxy guided by both the terraces and the step edges of the substrate, namely the dual-coupling mechanism [15] , [16] , [17] , [18] , [19] , [20] , [21] , [22] , [23] , [24] , [25] , [26] , [27] . However, numerous experimental observations showed that, in many cases, the atomic steps cannot guide epitaxial growth, even on the same kind of substrates. Currently, the epitaxy of non-centrosymmetric 2D materials can be achieved only in a very narrow experimental window. The decisive mechanism that ensures the epitaxy of non-centrosymmetric 2D materials remains elusive and is eagerly waiting to be fully explored. Here, we revealed that the accurate time sequence control of the simultaneous formation of grain nuclei and substrate steps is the key in the growth of single-crystal TMDs. Theoretical calculations reveal that the immature steps on the substrate promote grain nucleation near the step edges and guide the unidirectional alignment of 2D nuclei regardless of the step orientations. With this technique, unidirectionally aligned MoS 2 grains were achieved on sapphire (a, c, m, n, r and v planes with various step directions), MgO and rutile-TiO 2 substrates. This epitaxy was also demonstrated applicable to other TMDs like WS 2 , NbS 2 , MoSe 2 , WSe 2 and NbSe 2 . Our results reveal a robust mechanism for the universal growth of non-centrosymmetric 2D single crystals and thus would enhance the high-end applications of these 2D single crystals. Growth of unidirectionally aligned MoS 2 grains In this study, we show that the time sequence of 2D grain nucleation (t n ) and atomic step formation (t s ) on a substrate is the key factor that determines the success of epitaxy. Based on the sequence of t n and t s , the behaviour of 2D material growth is distinctly different: (i) if t n < t s or the nucleation of 2D grains occurs before the formation of the step edges, the growth is mainly controlled by the coupling between 2D grains and the substrate and the degeneracy of two antiparallel directions is not broken due to the lack of step edges (Fig. 1a ); (ii) if t n > t s or the nucleation of 2D grains occurs after the parallel step edges are formed, one must control the growth condition very carefully to ensure that all the grains nucleate at the step edges, and the epitaxial growth window is generally very narrow (Fig. 1b , such as special cutting angle, special steps direction and extremely high processing accuracy, and see Supplementary Tables 1 – 3 for details); (iii) t n ≈ t s or the nucleation of 2D grains occurs during the formation process of step edges, these immature step edges are active sites for the nucleation of 2D grains and the unidirectional alignment of the 2D grains is guaranteed in a broad growth window (Fig. 1c , such as high tolerance of substrates lattice structure, steps directions, types of substrate, and suitability of various TMDs growth, and see Supplementary Table 3 for details). Fig. 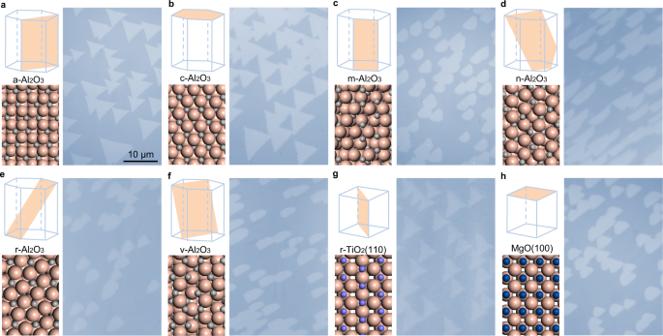Fig. 3: Universal growth of unidirectionally aligned MoS2grains on various substrates. Schematic diagrams of lattice structures of the substrates and optical images of MoS2grains grown on them. Unidirectionally aligned MoS2grains can be produced on a- (a), c- (b), m- (c), n- (d), r- (e), v-Al2O3(f), r-TiO2(110) (g), and MgO(100) surfaces (h). The orange, grey, violet and dark-blue spheres correspond to O, Al, Ti, and Mg atoms, respectively. The orange shaded planes in the lattice structures show the certain surface of the Al2O3, TiO2and MgO substrates. The scale bars for (a–h) are the same. 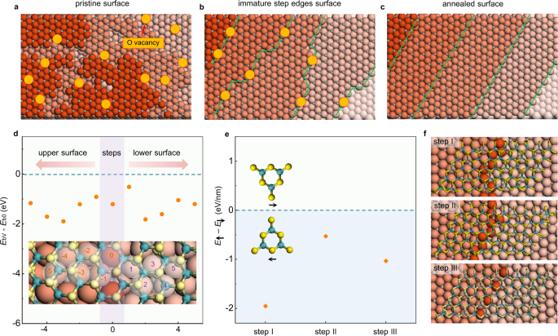Fig. 4: Mechanism of the simultaneous-formation-guided epitaxial growth of MoS2on vicinal c-Al2O3. a–cSchematic diagrams of the evolution of the c-Al2O3surface during annealing at high temperature.aThe original c-Al2O3surface is full of disorders and no clear separation of step edges and terraces.bDuring annealing, oxygen vacancies on terraces were gradually annealed, while some disorders, such as oxygen vacancies, still appeared in the blurred step edges.cAfter a long annealing time, the substrate is fully reconstructed with ultra-flat terraces separated by parallel step edges, and all the disorders on the substrate disappears. The red dotted circles represent the oxygen vacancy. The yellow, green, pink and grey spheres represent the S, Mo, O, and Al atoms, respectively. The green lines show the edges of the steps.dThe binding energy difference of a MoS2grain on a straight parallel step without O vacancy (Eb0) and on a defective step with different O vacancy at different sites (EbV). The negative values of (EbV–Eb0) reveals a stronger interaction between a MoS2grain and the defective steps. Inset: the different positions of O vacancy used in our calculations are marked by numbers and semi-transparent circles. The horizontal dashed line corresponds toEbV=Eb0. The light purple and light green shaded areas correspond to the steps and terrace areas.eEnergy difference between two antiparallel MoS2grains that cross three different types of step edges (I, II and III). The significant energy differences (0.5–2.0 eV/nm) show that all these step edges are able to break the symmetry of antiparallel MoS2grains on the c-Al2O3. All negative values imply that the alignment of the MoS2grain is not sensitive to the direction of the step edge and uni-alignment MoS2grains on various step edges can be formed. Inset: The positive and negative energy differences corresponding to the preferential of two antiparallelly aligned MoS2grains. The horizontal dashed line corresponds toE↑=E↓. The light blue and light green shaded area correspond toE↑<E↓andE↑>E↓, respectively.fThe MoS2grain on three types of step edges. 1: Growth of unidirectionally aligned MoS 2 grains by the simultaneous-formation-guided mechanism. a – c Schematic diagrams of the growth behaviour of non-centrosymmetric 2D grains when t n < t s ( a ), t n > t s ( b ) and t n ≈ t s ( c ). T n and t s are the 2D grains nucleation and atomic steps formation time, respectively. The shaded coloured areas represent the time window of t n and t s . The violet horizontal dashed lines represent the growth temperature. The yellow horizontal dashed lines correspond to the alignment probability of 1.0 and a certain value P. The growth window of 2D single crystals is greatly broadened when t n ≈ t s . d – g Atomic force microscopy (AFM) images of vicinal c-Al 2 O 3 surfaces annealed for different times (t s ). The steps are invisible for the original substrate ( d ) and are clear after long time annealing ( g ). 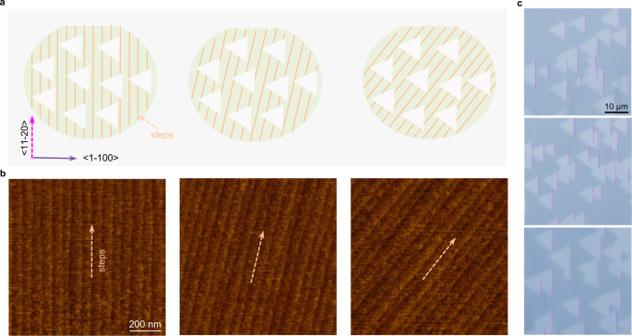e , f The pattern of step edges starts to appear at 50–60 min. h – j Optical images of MoS 2 grains on c-Al 2 O 3 at different nucleation times (t n ). Fig. 2: Growth of unidirectionally aligned MoS2grains on vicinal c-Al2O3with different step directions. aSchematic diagrams of MoS2grains on the surface with different step directions. The orange lines correspond to the parallel steps.bAFM images of the c-Al2O3surface. Different substrates exhibited different step directions.cOptical images of MoS2grains on Al2O3substrates shown in (b). One edge of all MoS2grains is along the <11–20> direction of Al2O3(calibrated by the cutting edge of the Al2O3wafer). The dashed fuchsia lines show parallel edges of MoS2grains. The scale bars in (b) and (c) are the same. 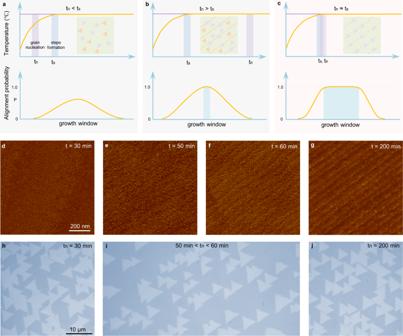Unidirectionally aligned MoS 2 grains were obtained when t n ≈ t s ( i ). Otherwise, antiparallel grains were produced ( h, j ). The scale bars in ( d – g ) and ( h – j ) are the same. Fig. 1: Growth of unidirectionally aligned MoS2grains by the simultaneous-formation-guided mechanism. a–cSchematic diagrams of the growth behaviour of non-centrosymmetric 2D grains when tn< ts(a), tn> ts(b) and tn≈ ts(c). Tnand tsare the 2D grains nucleation and atomic steps formation time, respectively. The shaded coloured areas represent the time window of tnand ts. The violet horizontal dashed lines represent the growth temperature. The yellow horizontal dashed lines correspond to the alignment probability of 1.0 and a certain value P. The growth window of 2D single crystals is greatly broadened when tn≈ ts.d–gAtomic force microscopy (AFM) images of vicinal c-Al2O3surfaces annealed for different times (ts). The steps are invisible for the original substrate (d) and are clear after long time annealing (g).e,fThe pattern of step edges starts to appear at 50–60 min.h–jOptical images of MoS2grains on c-Al2O3at different nucleation times (tn). Unidirectionally aligned MoS2grains were obtained when tn ≈ts(i). Otherwise, antiparallel grains were produced (h, j). The scale bars in (d–g) and (h–j) are the same. Full size image Figure 1d–g shows the step edge formation process on a vicinal Al 2 O 3 substrate. The pristine vicinal surface is rough and no clear pattern of step edges can be seen, which implies that both terraces and step edges are not well constructed (Fig. 1d ). During the annealing process, the pattern of step edges can be seen at ~50–60 min (Fig. 1e, f ), but the complete formation of parallel straight step edges requires additional ~150 min of annealing (Fig. 1g ). Thus, the time of the atomic step formation (t s ) can be determined to be 50–60 min under this annealing condition. Experimentally, the time of MoS 2 nucleation (t n ) can be controlled by the time of feeding the reactor with sulphur flux. We found that the epitaxy growth of unidirectionally aligned MoS 2 grains can be easily realized when t n ≈ t s , or by feeding the sulphur flux to the reactor during the step edge formation process (Fig. 1i and Supplementary Fig. 1 ). In contrast, feeding the sulphur either too early or too late (i.e., t n < t s or t n > t s ) always leads to a poor alignment of MoS 2 grains (Fig. 1h, j ). Systematic structural characterizations confirmed that once the unidirectionally aligned grains were realized, the parallel grains would seamlessly stitch into high-quality single-crystal films, consistent with all previous reports on graphene, hBN and TMDs [26] , [27] , [28] . The three-fold rotational symmetry of the low-energy electron diffraction (LEED) pattern (Supplementary Fig. 2 ) and the identical orientations of the polarized second-harmonic generation (SHG) pattern (Supplementary Fig. 3 ) confirmed the unidirectional alignment of MoS 2 grains grown on the vicinal c-plane sapphire (c-Al 2 O 3 ) surface and their seamless coalescences. The absence of any dark lines in the SHG mapping (Supplementary Fig. 4a, b ) or optical image of H 2 O-etched films (Supplementary Fig. 4c, d ) and the perfect crystalline lattices shown in the scanning transmission electron microscopic (STEM) images (Supplementary Fig. 5 ) demonstrated the single crystallinity of the MoS 2 films. Optical and electrical measurements also reveal that the as-grown MoS 2 films are of high quality. The circular helicity in the polarized photoluminescence (PL) spectrum is as high as 80% (Supplementary Fig. 6a, b ), which is competitive with exfoliated single-crystal MoS 2 flakes [29] . The full width at half maximum (FWHM) of the excitation peak is approximately 50 meV in the PL spectrum at room temperature (Supplementary Fig. 6c ), and the representative peak difference of A 1g and E 2g is ~19 cm −1 in the Raman spectrum (Supplementary Fig. 6d ), both suggesting that the samples are high-quality monolayer MoS 2 . We also fabricated field-effect transistor (FET) devices at different locations of single-crystal MoS 2 on 300 nm SiO 2 /Si substrates. The highest mobility reaches ~45 cm 2 (Vs) −1 and the average mobility is ~38 cm 2 (Vs) −1 measured at room temperature (Supplementary Figs. 7 , 8 ), which is also comparable to that of exfoliated ones [30] . Growth of MoS 2 on c-Al 2 O 3 with different step directions In previous growth of non-centrosymmetric 2D single crystals, such as h-BN and TMDs, the epitaxy requires atomic steps along a certain direction of the substrate and can only be realized on specially-designed substrates after tremendous experimental attempts [18] , [19] , [20] , [21] , [22] , [23] , [24] , [25] , [26] , [27] . Astonishingly, we observed that the unidirectional alignment of MoS 2 grains grown in our experiments can be realized on various vicinal Al 2 O 3 substrates regardless of the step orientations. We custom-fabricated vicinal c-Al 2 O 3 substrates with various cutting directions (Fig. 2a ) that determined the alignments of the step edges (Fig. 2b ). Among the 9 kinds of step directions we tested, all the grown MoS 2 grains were aligned along the <11–20> direction of the c-Al 2 O 3 surface (Fig. 2c and Supplementary Fig. 9 ). This result confirms the advantage of the previously proposed dual-coupling mechanism [27] , where the 2D materials epitaxy is guided by both the terraces and the step edges of the substrate: (i) the sapphire terrace-MoS 2 interaction leads to two preferred antiparallel orientations of the MoS 2 crystal and (ii) the sapphire step edge-MoS 2 interaction breaks the symmetry of the antiparallel orientations. This study further shows that the symmetry of the antiparallel aligned MoS 2 grains can be broken by step edges along different directions, which enables the epitaxial growth of various 2D materials on different substrates. Fig. 2: Growth of unidirectionally aligned MoS 2 grains on vicinal c-Al 2 O 3 with different step directions. a Schematic diagrams of MoS 2 grains on the surface with different step directions. The orange lines correspond to the parallel steps. b AFM images of the c-Al 2 O 3 surface. Different substrates exhibited different step directions. c Optical images of MoS 2 grains on Al 2 O 3 substrates shown in ( b ). One edge of all MoS 2 grains is along the <11–20> direction of Al 2 O 3 (calibrated by the cutting edge of the Al 2 O 3 wafer). The dashed fuchsia lines show parallel edges of MoS 2 grains. The scale bars in ( b ) and ( c ) are the same. Full size image Universal growth of MoS 2 on various substrates In addition to the vicinal c-plane Al 2 O 3 surface, we found that the current strategy for epitaxial growth of 2D single crystals is applicable for many other substrates. If the nucleation time matches the time of step edge formation well, unidirectionally aligned TMDs of different types can be easily grown on various substrates. As shown in Fig. 3a–h , the growth of unidirectionally aligned MoS 2 grains was realized on various vicinal a, c, m, n, r, and v planes of Al 2 O 3 , the vicinal rutile TiO 2 (110) surface and the vicinal MgO(100) surface (Supplementary Figs. 10 , 11 ). Once again, we noticed that the alignment of the MoS 2 grains does not depend on the step edge direction (Supplementary Figs. 12 , 13 ). Besides MoS 2 , we also realized the growth of unidirectionally aligned WS 2 , NbS 2 , MoSe 2 , WSe 2 and NbSe 2 grains (Supplementary Fig. 14 ). Thus, the epitaxial growth of non-centrosymmetric two-dimensional single-crystal metal dichalcogenides can be robustly achieved on many different substrates by initiating the TMDs growth during the step edge formation process. Fig. 3: Universal growth of unidirectionally aligned MoS 2 grains on various substrates. Schematic diagrams of lattice structures of the substrates and optical images of MoS 2 grains grown on them. Unidirectionally aligned MoS 2 grains can be produced on a- ( a ), c- ( b ), m- ( c ), n- ( d ), r- ( e ), v-Al 2 O 3 ( f ), r-TiO 2 (110) ( g ), and MgO(100) surfaces ( h ). The orange, grey, violet and dark-blue spheres correspond to O, Al, Ti, and Mg atoms, respectively. The orange shaded planes in the lattice structures show the certain surface of the Al 2 O 3 , TiO 2 and MgO substrates. The scale bars for ( a – h ) are the same. Full size image Mechanism of the simultaneous-formation-guided epitaxy To deeply understand the mechanism for the universal epitaxy, we performed theoretical analysis with density functional theory (DFT) calculations. Our study clearly showed that (i) the step edge is essential for breaking the centrosymmetry of the substrate for the epitaxial growth of two-dimensional single-crystal metal dichalcogenides and (ii) the strong interaction between the 2D material and the immature step edges during the annealing process ensures the initial nucleation of 2D grains near the step edges to break the equivalence of the antiparallel grains subsequently for unidirectional alignment. Taking MoS 2 growth on a vicinal c-Al 2 O 3 surface as an example, an as-cut Al 2 O 3 surface is generally full of disorders, where the step edges and terraces are randomly distributed and cannot be distinguished (Fig. 4a ). After long time annealing, the surface is fully reconstructed and ultra-flat terraces separated by parallel sharp step edges can be seen (Fig. 4c ). During the reconstruction process, most of the disorders, such as oxygen vacancies, on terraces are annealed but those near step edges are not (Supplementary Fig. 15 ) [31] , [32] , [33] , [34] . These immature step edges are expected to have many defects and thus are chemically active to ensure that the nucleation of most 2D grains occurs near step edges (Fig. 4b ). We calculated the binding energy of a MoS 2 near an oxygen vacancy. The results clearly showed that an oxygen vacancy can enhance the binding of a MoS 2 flake to the substrate by Δ E b ~1.0 eV (Fig. 4d ). We also compare the MoS 2 cluster nucleation on sapphire surface without steps, with perfect step edges, and with defective step edges, respectively (Supplementary Fig. 16 ). The result shows that the defective step edge apparently results in a stronger binding with MoS 2 compared to both flat terrace and perfect step edge. Especially, the binding energy continuous decreases with the increase of the number of O vacancies. Such a stronger binding leads to much easier TMD nucleation near the immature step edges. Therefore, the simultaneous formation of TMD nuclei and substrate steps guarantee most nucleation occurs around the step edges. Fig. 4: Mechanism of the simultaneous-formation-guided epitaxial growth of MoS 2 on vicinal c-Al 2 O 3 . a – c Schematic diagrams of the evolution of the c-Al 2 O 3 surface during annealing at high temperature. a The original c-Al 2 O 3 surface is full of disorders and no clear separation of step edges and terraces. b During annealing, oxygen vacancies on terraces were gradually annealed, while some disorders, such as oxygen vacancies, still appeared in the blurred step edges. c After a long annealing time, the substrate is fully reconstructed with ultra-flat terraces separated by parallel step edges, and all the disorders on the substrate disappears. The red dotted circles represent the oxygen vacancy. The yellow, green, pink and grey spheres represent the S, Mo, O, and Al atoms, respectively. The green lines show the edges of the steps. d The binding energy difference of a MoS 2 grain on a straight parallel step without O vacancy ( E b0 ) and on a defective step with different O vacancy at different sites ( E bV ). The negative values of ( E bV –E b0 ) reveals a stronger interaction between a MoS 2 grain and the defective steps. Inset: the different positions of O vacancy used in our calculations are marked by numbers and semi-transparent circles. The horizontal dashed line corresponds to E bV = E b0 . The light purple and light green shaded areas correspond to the steps and terrace areas. e Energy difference between two antiparallel MoS 2 grains that cross three different types of step edges (I, II and III). The significant energy differences (0.5–2.0 eV/nm) show that all these step edges are able to break the symmetry of antiparallel MoS 2 grains on the c-Al 2 O 3 . All negative values imply that the alignment of the MoS 2 grain is not sensitive to the direction of the step edge and uni-alignment MoS 2 grains on various step edges can be formed. Inset: The positive and negative energy differences corresponding to the preferential of two antiparallelly aligned MoS 2 grains. The horizontal dashed line corresponds to E ↑ = E ↓ . The light blue and light green shaded area correspond to E ↑ < E ↓ and E ↑ > E ↓ , respectively. f The MoS 2 grain on three types of step edges. Full size image Next, let’s consider the mechanism of unidirectional alignment of nucleated TMDs near step edges. Because of the C 2 symmetry of the c-Al 2 O 3 substrate, the couplings between a MoS 2 lattice and the c-Al 2 O 3 terrace lead to two equivalent antiparallel alignments of MoS 2 [25] . However, once the nucleation started near the step edges of a substrate, the equivalency between the antiparallel TMDs lattices could be broken and ensured the unidirectional alignment of MoS 2 grains (Fig. 4e, f ). Our calculations clearly show that the symmetry of the antiparallel aligned MoS 2 grains can be broken by step edges along different directions and the most stable alignment remains for a large variation in step edge directions. As shown in Fig. 4e, f , all three different step edges distinguish the antiparallel MoS 2 by ~1 eV/nm, and the preferred alignment is the same. In principle, this mechanism has broad applications for the growth of a variety of 2D materials on desired substrates, and thus is universal for the growth of 2D single crystals (calculations of WS 2 on c-Al 2 O 3 and WS 2 /MoS 2 on a-Al 2 O 3 are shown in Supplementary Fig. 17 ). Utilizing the full potential of 2D materials largely depends on the vertical integration of different single-crystal films [35] . At present, the transfer and integration techniques of 2D materials are very mature. However, the kinds of 2D single crystals that can be prepared on the wafer scale are very limited thus far. Our methodology opens an avenue to grow many kinds of 2D single crystals on desired substrates and will be very likely to proceed their integration for high-end electronic and optical applications. Detailed information of c-Al 2 O 3 Raw Material: 99,999%, High Purity, Monocrystalline Al 2 O 3 ; Growth Method: Kyropoulos; Crystal Grade: Optical Grade 1; Processing Grade: Epi-ready; Diameter: 50.8 mm + /− 0.1 mm; Thickness: 430 μm + /− 25 μm; Primary Flat Orientation A-plane (11–20) +/− 0.2°; Primary Flat Length: 16.0 mm + /− 1.0 mm; Front Surface: Epi-polished, Ra < 0.2 nm; Back Surface: Fine ground, Ra = 0.8 μm–1.2 μm. Growth of single-crystal MoS 2 monolayer on vicinal c-Al 2 O 3 MoS 2 monolayer grains and films were grown on unannealed Al 2 O 3 substrates (a, c, m, n, r, and v planes, Dongda Times (Chengdu) Technology Co., LTD) in a chemical vapour deposition (CVD) system with three temperature zones. S (Alfa Aesar, 99.9%) powder, MoO 3 (Alfa Aesar, 99.99%) powder and NaCl (Greagent, 99.95%) mixture, Al 2 O 3 were placed on the upstream end of the quartz tube, temperature zone-I and temperature Zone-III of the tube furnace, respectively. During the growth process, under a mixed gas flow (Ar, 30 sccm; H 2 , 0–5 sccm), the temperature zone-I, II and III of the tube furnace were heated to 565, 850, and 975 °C within 50 min, respectively. During this process, the sapphire substrate would start construct and the immature steps started to appear. When zone-I was heated to 400 °C, the S (Alfa Aesar, 99.9%) powder was heated to 150 °C, within 15 min by a heating belt. When zone-I was heated to 510 °C, a little amount of oxygen was introduced. The growth time was 10–40 min to obtain MoS 2 grains or films. After the growth, the system was naturally cooled to room temperature with 300 sccm Ar. The detailed growth setup and temperature ramps can be seen in Supplementary Fig. 18 . Growth of WS 2 , NbS 2 , MoSe 2 , WSe 2 and NbSe 2 on vicinal c-Al 2 O 3 The growth recipes were very similar to that for MoS 2 except for the replacement of MoO 3 by WO 3 or Nb 2 O 5 source, S by Se source and the temperature settings were adjusted accordingly. During WS 2 growth, the temperature of the S source, zone-I, II, III, were set as 150, 645, 850, and 975 °C under gas flow (Ar, 30 sccm). During NbS 2 growth, the temperatures were set as 150, 745, 850, and 965 °C. During MoSe 2 growth, the temperatures were set as 250, 565, 850, and 975 °C. During WSe 2 growth, the temperatures were set as 250, 645, 850, and 975 °C. During NbSe 2 growth, the temperatures were set as 250, 745, 850, and 965 °C. Characterization (i) LEED measurements were performed using Omicron LEED system in UHV with base pressure < 3 × 10 −7 Pa. AFM measurements were performed using Bruker Dimensional ICON under atmospheric environment. (ii) Optical measurements. Optical images were conducted with an Olympus microscope (Olympus BX51). Raman spectra were obtained with a home-made Raman system with laser excitation wavelength of 532 nm and power of ~0.5 mW. Low-temperature PL spectra were obtained at 15 K using a home-made optical cryostat with laser excitation wavelength of 532 nm and power of ~8 μW. Polarized light was generated with a super-achromatic quarter-wave plate (Thorlabs SAQWP05M-700) and the photoluminescence was analysed through the same quarter-wave plate and a linear polarizer. SHG mapping was obtained using the same system under excitation from a femtosecond laser centred at 820 nm with average power of 800 μW (Spectra-Physics Insight system with pulse duration of 100 fs and repetition rate of 80 MHz). (iii) TEM characterization. The MoS 2 sample were transferred onto homemade monolayer graphene TEM grids using the polymethyl-methacrylate-based transfer technique. Graphene TEM grids were made by transferring large-area monolayer single-crystal graphene on commercial holey carbon TEM grids (Zhongjingkeyi GIG-2010-3C). STEM experiments were performed in FEI Titan Themis G2 300 operated at 80 kV. (iv) Device fabrications and measurements. The FETs were fabricated through standard microfabrication process by electron beam lithography techniques. The MoS 2 sample was transferred from sapphire substrate by wet method assisted by KOH solution (1 Mol/L, 110 °C). The Bi/Au contact electrodes (~10/30 nm) were fabricated by e-beam deposition system with a low vacuum ~3 × 10 −7 Pa. All the electrical measurements were carried out in a Janus probe station (base pressure 10 −6 Torr) with Agilent semiconductor parameter analyser (B1500, high resolution modules) at room temperature. Computational details Geometric optimization and energy calculations of the MoS 2 /c-Al 2 O 3 systems were carried out using density functional theory (DFT) as implemented in Vienna Ab-initio Simulation Package. The generalized gradient approximation (GGA) with the Perdew–Burke–Ernzerhof (PBE) exchange-correlation function was used with the plane-wave cutoff energy set at 400 eV for all calculations. The dispersion-corrected DFT-D 3 method was used because of its good description of long-range vdW interactions for multi-layered 2D materials. The geometries of the structures were relaxed until the force on each atom was less than 0.01 eV Å −1 , and the energy convergence criterion of 1 × 10 −5 eV was met. The Al 2 O 3 surfaces were modelled by a periodic slab and some bottom layers were fixed to mimic the bulk, a 1 × 1 × 1 Monkhorst–Pack k-point mesh was adopted. The binding energies of the MoS 2 – substrate hybrid, namely, E b = ( E hyb – E MoS2 – E sub )/S, was calculated using the relaxed structures, where E hyb is the total energy of the hybrid; E MoS2 and E sub represent the energies of MoS 2 and the substrate, respectively; and S is the area of the MoS 2 cluster. To estimate the Al 2 O 3 step–MoS 2 interaction, two antiparallel MoS 2 nanoribbons with a length of about 1.6 nm were placed on the steps of the c-Al 2 O 3 surface and then relaxed. The energy difference was defined as ΔE = E ↑ – E ↓ , E ↑ = E 1 /L and E ↓ = E 2 /L, where E 1 and E 2 are the total energies of the hybrid system, respectively, and L is the length of the nanoribbon. Similar calculations were also conducted for the MoS 2 /a-Al 2 O 3 systems.